A 2,000-year reconstruction of the rain-fed maize agricultural niche in the US Southwest Humans experience, adapt to and influence climate at local scales. Paleoclimate research, however, tends to focus on continental, hemispheric or global scales, making it difficult for archaeologists and paleoecologists to study local effects. Here we introduce a method for high-frequency, local climate-field reconstruction from tree-rings. We reconstruct the rain-fed maize agricultural niche in two regions of the southwestern United States with dense populations of prehispanic farmers. Niche size and stability are highly variable within and between the regions. Prehispanic rain-fed maize farmers tended to live in agricultural refugia—areas most reliably in the niche. The timing and trajectory of the famous thirteenth century Pueblo migration can be understood in terms of relative niche size and stability. Local reconstructions like these illuminate the spectrum of strategies past humans used to adapt to climate change by recasting climate into the distributions of resources on which they depended. Humans experience, adapt to and influence climate at local scales. Recent paleoclimate research, however, tends to focus on continental, hemispheric or global scales, making it difficult for archaeologists and paleoecologists to study local effects of past climate change. Furthermore, studies that have attempted high-resolution climate-field reconstruction [1] , [2] , [3] , [4] have generally failed to recast climate into the distributions of resources on which humans depend, such as viable land for agriculture and crop productivity. Regional- to local-scale paleoclimate reconstructions from tree-ring (t-r) chronologies have been typically generated using one of two basic methods. Well-known regional [5] and climate field [1] , [2] , [3] reconstructions of drought employ principal component regression (PCR) in an effort to calibrate the joint variance in a set of t-r chronologies to a given regional or locally interpolated climate signal. In contrast, researchers primarily interested in local climate tend to select one or a few local t-r chronologies for calibration to a local climate signal, either using ordinary least squares linear regression [6] or, less commonly, mean-variance matching [7] or PCR on a limited selection of chronologies [8] , [9] . Researchers have long noted that certain species of trees in particular ecological settings are better or worse at predicting a given climate signal [10] , and many methods employ expert knowledge about these proxy/climate relationships [11] or else screen potential t-r chronologies using basic correlation statistics [1] , [12] . State-of-the-art, compute-intensive methods such as BARCAST [4] approach paleoclimate reconstruction in a fundamentally different and promising way—by simultaneously endogenizing the spatiotemporal covariance structure of both empirical climate measurements and climate proxy data—but to our knowledge these have not yet been attempted on very high-resolution (<1 km) spatiotemporal fields. Both the data-laden principal component techniques and the more selective manual methods illustrate the careful balancing act undertaken by those attempting local paleoclimate reconstruction: We know that such reconstructions require focus on local conditions (which we expect will be proxied by local t-r chronologies), but we also recognize that our paleoclimate inferences are strengthened when patterns are robust across available chronologies. We seek a method that not only emulates well-informed manual selection of t-r chronologies for local climate reconstruction, but also automates the discovery of proxies causally linked to the climate signal, which may not have been considered by the researcher. For example, climate teleconnections may make non-local chronologies good proxies for local conditions in some circumstances. Here we address both the need for improved climate-field reconstruction methods and the need for reconstructions relevant to human experience and adaptation. We generate 2,000-year reconstructions of net water-year precipitation and accumulated heat over the growing season for two large and environmentally heterogeneous areas (the ‘VEPIIN’ and ‘VEPIIS’ study areas; Fig. 1 ) in the southwestern United States (SWUS) with very dense populations of prehispanic maize ( Zea mays ) farmers. We then recast these reconstructions as estimates of the rain-fed maize growing niche across the regions. By doing so, we are able to assess the degree to which significant cultural transitions in the Ancestral Pueblo SWUS can be explained by changes in the spatial distribution of the niche. We find niche size and stability to be highly variable within and between the regions. Prehispanic rain-fed maize farmers in both regions tended to live in agricultural refugia—areas most reliably in the rain-fed agricultural niche. Also, both the timing and trajectory of the famous thirteenth century Pueblo migration in the region can be understood in terms of the relative niche size and stability in the two regions. Local reconstructions similar to those presented here illuminate the spectrum of strategies past humans and other organisms used to adapt to climate change by recasting climate into the distributions of resources on which species depend. 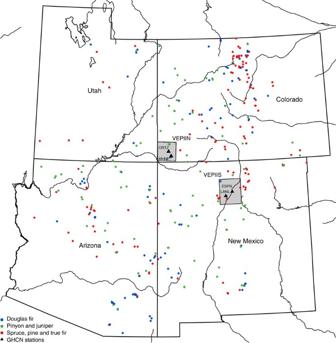Figure 1: The Four Corners region of the southwestern United States. Tree-ring chronologies are coloured dots, our two study areas are shown as grey rectangles and weather stations used for model comparison (Supplementary Methods) are shown as black triangles. MVNP, Mesa Verde National Park, Colorado; CRTZ, Cortez, Colorado; LANL, Los Alamos National Laboratory, New Mexico; ESPN, Española, New Mexico. Figure 1: The Four Corners region of the southwestern United States. Tree-ring chronologies are coloured dots, our two study areas are shown as grey rectangles and weather stations used for model comparison ( Supplementary Methods ) are shown as black triangles. MVNP, Mesa Verde National Park, Colorado; CRTZ, Cortez, Colorado; LANL, Los Alamos National Laboratory, New Mexico; ESPN, Española, New Mexico. Full size image Climate-field reconstruction We employ a variable ranking and selection method developed in quantitative genomics called CAR (Correlation-Adjusted corRelation) regression [13] . The CAR method was developed as a robust variable-ranking method for ill-posed inference problems, where the number of variables is much larger than the number of observations. Such high-dimensional problems are typical in paleoclimate reconstruction, where the number of available annually resolved climate proxies continues to rapidly expand, but observed climate data are generally limited to the last century or so. The CAR method first orthagonalizes the t-r chronologies over a historic calibration period using the Mahalanobis transform [13] . It then ranks the orthogonal chronologies by their squared correlations with the observed climate signal. Ranked chronologies are then added step-wise into a linear regression until cross-validated root mean squared prediction error (RMSE) is minimized. The CAR method is similar to principal component techniques. Accounting for covariance between predictors (in this case, t-r chronologies), the method determines which linear combination of chronologies best predicts a given climate signal. Unlike PCA, although, the CAR method explicitly ranks and selects chronologies based on the mutual information shared between the t-r chronologies and the climate signal. Using an associated shrinkage regression technique [14] , [15] , we then generate unique and highly accurate reconstructions across a spatiotemporal climate field. We generate spatiotemporal reconstructions by first performing independent CAR reconstructions for each of 17,554 grid cells in our two study areas (see Methods). Starting with the calibration period (1924–1983), for each cell and each climate signal, we use CAR ranking to select the best linear combination of t-r chronologies, then generate a retrodiction using those chronologies extending back in time as far as their joint duration allows. At that point, we calibrate a new model using the remaining available chronologies. We repeat this process until the retrodiction reaches the date of initial interest, AD 1. Finally, to remove spatial artefacts inherent to the discrete nature of the CAR proxy selection procedure, the reconstructions are spatially standardized such that for any given year all cells in a study area are using the union of all the selected sets of t-r chronologies in their reconstructions. 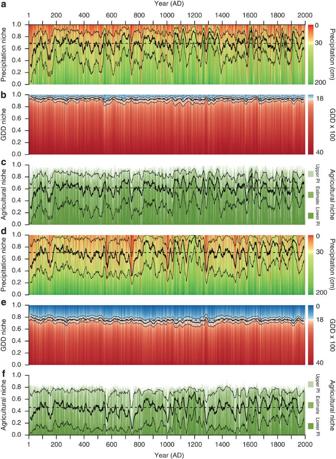Figure 2: The rain-fed maize agricultural niche through time. Each year is represented by the cumulative proportion of the landscape at different values, represented by colour gradients defined in the right margin. The colour gradient of each panel breaks at the extent of that signal’s agricultural niche. The thick solid line in each panel is a 21-year running mean of the estimated proportion in each niche; the thin solid lines are the upper and lower prediction intervals (see Methods); the dashed line is the mean estimated proportion in the niche over the entire reconstruction. (a) VEPIIN net water-year precipitation, green portion in niche. (b) VEPIIN growing-season growing degree days (GDDs), red portion in niche. (c) VEPIIN rain-fed maize agricultural niche, light green in niche upper PI, medium green in niche estimate, dark green in niche lower PI. (d–f) The same asa–cfor the VEPIIS study area. Figure 2 presents a summary of the spatiotemporal paleoclimate reconstructions as the cumulative proportion of the landscape at different climate values, through time; Supplementary Movie 1 presents the actual climate field reconstructions. As is typical of climate in the SWUS, summer precipitation and growing-season growing degree days (GDDs) are negatively correlated at most locations. GDD shows less year-to-year variation than does precipitation. Precipitation reconstructions for both study areas show general agreement with other regional reconstructions of drought [3] , [16] ; major pan-regional drought episodes occurred in the first half of the first century AD, the mid-AD 100s, mid-AD 700s, late AD 1200s and late AD 1500s. Several major droughts affect the VEPIIS area more strongly than the VEPIIN area, including those around AD 1000, the mid-AD 1100s and the late AD 1400s. Figure 2: The rain-fed maize agricultural niche through time. Each year is represented by the cumulative proportion of the landscape at different values, represented by colour gradients defined in the right margin. The colour gradient of each panel breaks at the extent of that signal’s agricultural niche. The thick solid line in each panel is a 21-year running mean of the estimated proportion in each niche; the thin solid lines are the upper and lower prediction intervals (see Methods); the dashed line is the mean estimated proportion in the niche over the entire reconstruction. ( a ) VEPIIN net water-year precipitation, green portion in niche. ( b ) VEPIIN growing-season growing degree days (GDDs), red portion in niche. ( c ) VEPIIN rain-fed maize agricultural niche, light green in niche upper PI, medium green in niche estimate, dark green in niche lower PI. ( d – f ) The same as a – c for the VEPIIS study area. Full size image Niche reconstruction Climate change affects human behaviour in many ways, but in agrarian societies such as the prehispanic Pueblo peoples inhabiting these two study areas—who derived ~70% of their dietary biomass from maize [17] —its most direct influence is on agricultural productivity. Therefore, we convert our paleoclimate reconstructions into estimates of the spatial extent of the rain-fed maize agricultural niche within each landscape. We model agricultural niche—as opposed to modelling productivity directly for a particular landrace of maize [8] , [9] —as an acknowledgement of the phenotypic plasticity of maize that allows for rapid adaptation to changing local conditions [18] . We seek to answer the question: Given ample time and human effort, where on the landscape could we reasonably expect locally adapted maize landraces to flourish? Accordingly, we threshold the niche at the 30-cm isohyet for the net water-year precipitation reconstruction, which Shaw [19] and others [20] take as the lower bound for rain-fed maize cultivation; and we threshold the niche at 1,800 GDD (measured in Fahrenheit GDDs) for the growing-season GDD reconstruction, following experimental estimates for ancestral landraces [21] , [22] and previous reconstructions [20] . For each year, we define the rain-fed maize agricultural niche as the portion of the landscape that satisfies both of these thresholds ( Fig. 3 ). 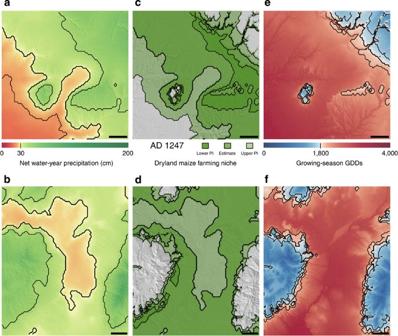Figure 3: The rain-fed maize agricultural niche in AD 1247. The upper panels represent the VEPIIN study area; the lower panels represent VEPIIS. Each panel’s colour gradient breaks at the extent of that signal’s agricultural niche. Thin black lines are at the upper and lower prediction intervals. Scale bar: 10 km. (a,b) Net water-year precipitation, green portion in niche. (e,f) Growing-season GDDs, red portion in niche. (c,d) The rain-fed maize agricultural niche, light green portion in upper PI, medium green portion in niche, dark green portion in lower PI.Supplementary Movie 1presents the full 2,000-year reconstruction. Figure 3: The rain-fed maize agricultural niche in AD 1247. The upper panels represent the VEPIIN study area; the lower panels represent VEPIIS. Each panel’s colour gradient breaks at the extent of that signal’s agricultural niche. Thin black lines are at the upper and lower prediction intervals. Scale bar: 10 km. ( a , b ) Net water-year precipitation, green portion in niche. ( e , f ) Growing-season GDDs, red portion in niche. ( c , d ) The rain-fed maize agricultural niche, light green portion in upper PI, medium green portion in niche, dark green portion in lower PI. Supplementary Movie 1 presents the full 2,000-year reconstruction. Full size image Niche size and stability are highly variable within and between the two regions ( Figs 2 and 3 ). The niche reconstructions are primarily driven by high-amplitude changes in the size of the precipitation niche in both areas, and although cold periods do impact higher-elevation locations they usually co-occur with an increase in precipitation across the landscape ( Supplementary Movie 1 ). The proportion of the landscape available for rain-fed maize cultivation is generally much less in the VEPIIS study area than in the VEPIIN, primarily due to elevation differences in the two regions. Ancestral Pueblo demographic transitions We can more directly compare the two regions by analysing the deviation of each niche-series from its 2,000-year mean and thus assessing push- and pull-factors that might have stimulated population flows between the regions ( Fig. 4 ). Here we focus on the period salient to the Prehispanic Pueblos (AD 500—AD 1500). The VEPIIN study area outperforms the VEPIIS study area for much of the initial settlement of maize agriculturalists in VEPIIN (AD 600—AD 750) [23] . The pan-regional drought in the mid-AD 700 s is substantially worse and occurs over a longer duration in the southern area than in the north, and may partially explain the relatively late expansion of maize farmers in the northern Rio Grande, which accelerates after AD 750 (ref. 24 ). In contrast, the VEPIIS study area outperforms the VEPIIN area from just after the mid-AD 1100s drought through the mid-AD 1200s. During this same time Pueblo emigration began from the northern SWUS in general, and likely from VEPIIN in particular [25] , with the northern Rio Grande one of the most important destinations [26] . 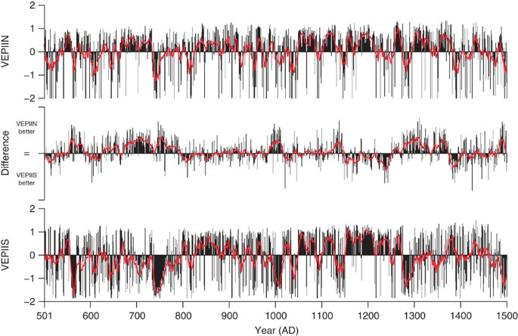Figure 4: The difference in niche size between the study areas. The top and bottom plots present the standardized proportion of each landscape in the niche and the centre plot presents the difference between the two study areas during AD 501—AD 1500. The red line in each panel is a 11-year running mean of the series. The centre plot takes the difference of the upper and lower plots. Figure 4: The difference in niche size between the study areas. The top and bottom plots present the standardized proportion of each landscape in the niche and the centre plot presents the difference between the two study areas during AD 501—AD 1500. The red line in each panel is a 11-year running mean of the series. The centre plot takes the difference of the upper and lower plots. Full size image Locating ancestral Pueblo agricultural refugia Spatial analysis of niche stability reveals the location of refugia during agricultural downturns ( Fig. 5 ). In the VEPIIN study area, much of the Mesa Verde cuesta is in the niche more than 90% of years over the last two millennia, and the northeast half of the Montezuma Valley—the region of modern rain-fed bean farming—is in the niche more than 80% of years. The region of the McElmo Dome surrounding Sand Canyon and Goodman Point, two of the largest villages during the late AD 1200s (ref. 27 ), is also in the niche more than 80% of years. In the VEPIIS study area, much of the Pajarito Plateau on the eastern flanks of the Jemez mountains is in the niche more than 90% of years. This portion of the VEPIIS study area experienced more immigration in the AD 1200s and early AD 1300s than any other part of VEPIIS [26] . Rain-fed maize agriculturalists apparently settled first on the portion of the landscape most suitable to rain-fed maize agriculture; only later did they start developing and adopting the water management technology and mobility strategies required to farm elsewhere in the region [7] , [28] . Our reconstruction of the maize niche in VEPIIS differs from other reconstructions of precipitation for northern Rio Grande [29] in that ours identifies the late 1200s as a period of significant drought in the region. As a refugium in times of drought, the Pajarito Plateau would therefore have been particularly attractive for people arriving from the north at that time. 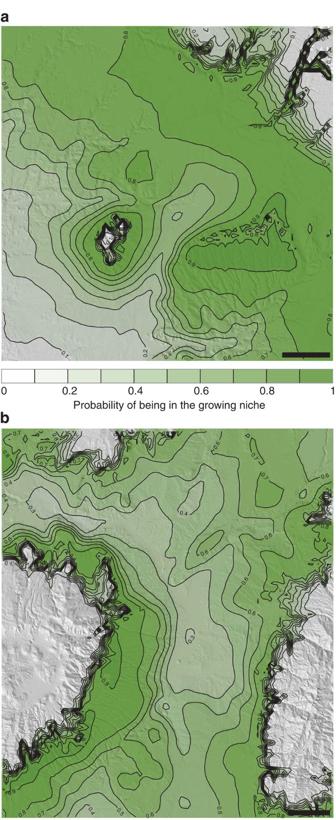Figure 5: Ancestral Pueblo agricultural refugia. These maps show the proportion of years (AD 1–2000) each location is in the rain-fed maize agricultural niche. More shaded areas are in the niche more often. In the VEPIIN study area (a), the Mesa Verde cuesta (lower-right quadrant) is in the niche more than 90% of the years in the last two millennia. In the VEPIIS area (b), portions of the Pajarito Plateau (lower-left quadrant) are also in the niche more than 90% of the years. Scale bar, 10 km. Figure 5: Ancestral Pueblo agricultural refugia. These maps show the proportion of years (AD 1–2000) each location is in the rain-fed maize agricultural niche. More shaded areas are in the niche more often. In the VEPIIN study area ( a ), the Mesa Verde cuesta (lower-right quadrant) is in the niche more than 90% of the years in the last two millennia. In the VEPIIS area ( b ), portions of the Pajarito Plateau (lower-left quadrant) are also in the niche more than 90% of the years. Scale bar, 10 km. Full size image The reconstruction presented here suggests where Pueblo people may have been able to practice rain-fed maize agriculture, but not how productive their efforts may have been. More nuanced analyses of CAR-based paleoclimate reconstructions—such as cropping system models accounting for adaptation of maize landraces to local conditions [18] and integrating soils data [20] and killing degree days [18] —will improve our understanding of how humans and their domesticates adapted to changing climate conditions. Our paleoclimate reconstructions can also be improved by better accounting for low-frequency temperature change, perhaps via a regionalized application of wavelet modulation with pollen and speleothem data [30] , [31] . Temperature anomalies of the scale of the Medieval Warm Period and Little Ice Age in North America (each within ±1° Celsius from the long-term average [31] ) may have had a substantial impact on GDD in our region. A 1°-Celsius decrease in average growing-season temperature would result in an approximately 275 GDD decrease (in Fahrenheit GDDs), effectively shutting down high-elevation maize production in areas like the Mesa Verde cuesta. Local, low-frequency temperature reconstructions have not yet been attempted at the scale of our subregions, however, so it is an open question as to whether the effects of regional climate anomalies were consistent across regions. From our high-frequency results, neither of these major climate anomalies appears to have had a substantial impact on precipitation. Compute-intensive methods like the one presented here may be used to discover new ecological knowledge, both about landscapes themselves and about causal connections between climate and climate proxies. A complete exploration of the ecological ramifications of our paleoenvironmental reconstruction is beyond the scope of this study, but several initial observations may be made. Water-year precipitation in VEPIIN is best reconstructed using pinyon, juniper and Douglas fir chronologies from the western slope of the Colorado Rocky Mountains. In contrast, the precipitation system in VEPIIS is dominated by the summer-arriving North American Monsoon, which is connected to precipitation intensity in southern Arizona and throughout southern and central New Mexico [32] , [33] , [34] . The majority of chronologies selected for precipitation reconstruction in VEPIIS are low- and mid-elevation chronologies from southern Arizona and New Mexico. Tree-ring chronologies selected for growing-season GDD reconstructions are much more similar between the landscapes; chronologies are generally selected from among higher-elevation spruces, pines, true firs and Douglas firs, and the chronologies selected are often more distant than for precipitation. Future research might focus on identifying ecological zones by their common selected proxies, and the temporal consistency of relationships between proxies. The archaeological and paleoecological record provide important information about how humans and other organisms have adapted to past climate change, and how they might adapt in the future. Regardless of contemporary technological innovations, humans and other species struggle to adapt to climate change on the timescales and amplitudes present in both our reconstructions and contemporary projections. The rate and scale of contemporary climate change are unprecedented at a hemispheric level; however, past agrarian populations have had to adapt to rapid, dramatic changes in their local environments. Archaeological knowledge—analysed in the context of reconstructed environments—is essential in understanding the dynamics and operation of coupled human and natural systems [35] . The experience in the Ancestral Pueblo SWUS suggests that, when faced with changing environments, humans will first seek alternative habitats that do not require them to change behaviour—such as the Pajarito Plateau—and only once those are unavailable will they develop or adopt alternative strategies. Generalizing to modern times, when confronted with rapidly changing environmental conditions, we should (i) identify those environmental niches that will remain open or even improve because of rapid climate change, and (ii) identify regions where contemporary strategies simply will not work given climate predictions, so that alternative strategies may be more rapidly adopted. Assessing either of these requires accurate, precise and local reconstructions of how resource distributions change in response to climate change. Study areas The study areas in this analysis are drawn from the Village Ecodynamics Project (VEP), a research initiative investigating long-term relationships between humans and the environment in the SWUS [36] , [37] ( Fig. 1 ). The first study area (VEPIIN) is a 4,600 km 2 region in southwestern Colorado encompassing Mesa Verde National Park, Canyons of the Ancients National Monument, the Montezuma Valley, portions of the Ute and La Plata piedmonts, and the contemporary towns of Cortez, Dolores, and Mancos, Colorado. The area is defined in NAD83, Zone 12 Universal Transverse Mercator grid units; it extends from 672,800 m E to 740,000 m E, and 4,102,000 m N to 4,170,000 m N. The second area (VEPIIS) is a 6,955 km 2 region in north-central New Mexico encompassing Pajarito Plateau, Bandelier National Monument, the Rio Grande and Chama river valleys, and the contemporary cities of Santa Fe, Los Alamos and Española, New Mexico. It extends from 359,200 m E to 435,800 m E, and 3,939,600 m N to 4,030,400 m N in NAD83, Zone 13 Universal Transverse Mercator coordinates. The climate reconstructions presented here were calculated on slightly larger areas than these study regions to account for spatial projection and resolution differences between the VEP regions and the Parameter-elevation Relationships on Independent Slopes Model (PRISM) interpolated climate data presented below. Tree-ring chronologies We used publicly available, standardized, pre-processed t-r chronologies in the International Tree-Ring Data Bank as of January 2014 (refs 38 , 39 ), that is, those without a trailing ‘A’ or ‘R’ in their file name). We downloaded all available chronologies and imported *.crn files into R using the dplR library [40] . We only retained chronologies that are from the United States of Arizona, Colorado, New Mexico and Utah, and that fully overlapped our calibration/validation period of 1924–1983 ( n =205); many long chronologies in the SWUS only extend to the early 1980s. Figure 1 shows the location and species information for the chronologies used in this study, and Fig. 6 shows the number of chronologies available through time. The length and availability of t-r chronologies are quite variable across records and species. Inclusion of chronologies updated more recently (but not yet in the International Tree-Ring Data Bank) would undoubtedly improve the skill of these reconstructions. 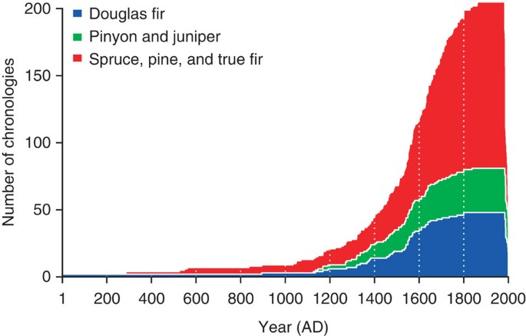Figure 6: Tree-ring chronology availability. Colours represent species classification. During the 1924–1983 calibration period 205 chronologies available. Figure 6: Tree-ring chronology availability. Colours represent species classification. During the 1924–1983 calibration period 205 chronologies available. Full size image Historic climate data We use the ~800 m-resolution PRISM interpolated monthly data grids (the ‘LT81m’ dataset) available from the Oregon State University [41] , [42] to calibrate annual reconstructions of water-year precipitation and growing-season GDDs. We calibrate our reconstruction to years 1924–1983. We follow Stahle and colleagues [6] in defining the water-year in the US Southwest as the previous October—current September, and we define the growing season as May—September of the current year. Monthly precipitation totals were summed over the water year. Growing season GDD was estimated by first calculating monthly GDD from monthly mean maximum and minimum temperatures using equation 1 (below), summed over the number of days for each month. May—September monthly GDD estimates were then summed to estimate net GDD for the growing season. All GDD results reported here are in Fahrenheit heat units; GDDs were converted from Celcius heat units to Fahrenheit heat units by multiplying by a factor of 1.8. The equation for daily GDD is: where T MAX is the maximum daily temperature, T MIN is the minimum daily temperature and T BASE is the temperature below which plant growth ceases, which we take to be 10 °C for maize. Here we use a series of corrections to equation (1) typically applied for calculating maize GDD [43] , which down-corrects T MAX and T MIN to an upper threshold ( T UT , here 30 °C) above which corn growth does not appreciably increase, and up-corrects T MAX and T MIN if they fall below T BASE (here 10 °C). To summarize: Net water-year precipitation and GDD grids were calculated for each of our two study areas. The VEPIIN study area includes 7,144 grid cells at 30 arc-s (~800 m) resolution. The VEPIIS study area includes 10,400 cells at the same resolution. Mean temperature in the Northern Hemisphere has trended dramatically upward over the twentieth century, potentially confounding reconstructions because of non-stationarity in the PRISM-based GDD calibration data [44] . We therefore tested whether these data show similar trends. Local to our study areas, the seasonal PRISM data for GDD are second-order stationary over the 1924–1983 period (although GDD trend higher post-1983). We performed the Priestley–Subba Rao test of non-stationarity [45] , [46] on each of the grid cells in each landscape ( Supplementary Fig. 1 ). None of the cells in either landscape have Priestley–Subba Rao P -values low-enough to reject the null hypothesis of stationarity at the P <0.05 level. This does not remove the possibility that past climate was non-stationary. Rutherford and colleagues found that reconstructions of non-stationary (forced) climate using a stationary calibration signal tend to underestimate reconstructed trends [44] . We attempt to compensate for this by performing mean and variance matching over the calibration period (below); however, our reconstructions should be considered conservative estimates of past low-frequency climate variability. Local reconstruction overview For each location (cell) in the PRISM data and each climate signal (water-year precipitation and growing-season GDD), we de-correlate the matrix of t-r chronologies by applying the Mahalanobis transform, using a Stein-type shrinkage approximation of the covariance matrix following [13] , [47] ; generate estimates of the marginal correlations between the training data and each decorrelated t-r chronology (the CAR scores); rank the t-r chronologies by their squared CAR scores; select the optimal set of t-r chronologies for use in a linear model by minimizing average RMSE over a threefold consecutive cross-validation, and estimate linear regression coefficients; standardize the set of chronologies to the union of the selected chronologies across all cells in each study area; retrodict the signal over the joint duration of the selected t-r chronologies; transform and scale the retrodiction such that the mean and variance of the retrodiction over the calibration period matches the mean and variance of the climate signal over the same period; repeat the preceding steps, going back through time as fewer t-r chronologies become available (see Fig. 6 ). Variable ranking by CAR score The CAR score is defined as the correlation between the outcome variable (in this case, water-year precipitation or growing-season GDD) and the Mahalanobis de-correlated predictors (the t-r chronologies) (ref. 13 [13] , page 11). The Mahalanobis transform is similar to other matrix orthogonalization methods, however, Zuber and Strimmer note that it is particularly desirable for variable selection in that it generates orthogonal variables that are nearest to and informative of the original standardized variables (ref. 13 [13] , pages 9–10). CAR scores reduce to raw correlations between the outcome and predictor variables as correlation among predictor variables vanishes (ref. 13 [13] , page 8). Furthermore, predictors that are highly correlated will have nearly identical CAR scores, leading to their co-selection (or co-rejection) when CAR scores are used in variable ranking and selection (ref. 13, page 13). Here we calculated CAR scores using the carscore method in the care package for R , developed by Zuber and Strimmer [47] . Because the number of available t-r chronologies (predictor variables) is larger than the number of observations (years in our calibration period, 1924–1983), we use estimate the correlation and covariance matrices using Stein-type shrinkage estimators [14] , [47] . The shrinkage intensity variables λ c and λ υ —the shrinkage intensities of the correlation and covariance matrices, respectively—were estimated for each cell using the complete set of 205 available t-r chronologies. Once CAR scores are calculated for each cell and each climate signal, t-r chronologies are ranked by their squared CAR scores. Variable selection by minimized RMSE There are many ways one could select variables once they are ranked, including removing null variables using an adaptive threshold [48] , optimized selection using compute-intensive cross-validation or classic model selection using information criteria such as Akaike’s Information Criterion [49] . Here we follow the suggestion of Zuber and Strimmer [13] and use threefold consecutive cross-validation over the 1924–1983 period to choose the set of t-r chronologies that minimizes RMSE, as well as to provide estimates of prediction error along our reconstructions. Spatial artefacts and chronology standardization The CAR reconstruction method—like all t-r-based paleoclimate reconstructions—assumes covariance relationships between the t-r chronologies in the calibration period remain consistent as the chronologies extend back in time. This ‘uniformitarian principle’ underlies all paleoclimate proxy research. Random signal noise in each t-r chronology causes these relationships to weaken at short timescales. This reality has required a variety of complex accommodations by paleoclimate researchers, from standardization using principal components as in the North American Drought Atlas [1] , [2] , [3] to explicitly accounting for inconsistencies in both the proxy and instrumental data using compute-intensive estimation of the spatial covariance and temporal evolution of the climate field in a hierarchical Bayesian framework [4] . Our reconstructions—when done with unique spatiotemporal combinations of locally CAR-selected chronologies—are affected by these issues as well. Locations on the landscape that are proximate to one another tend to select the same chronologies, and thus consistent spatial covariance between the locations is maintained. However, sometimes adjacent grid locations select a slightly different set of chronologies. When the covariance between the uniquely selected sets of chronologies breaks down, spatial artefacts occur such that usually smooth temperature and precipitation gradients become coarse and step-like. Panels (a) and (b) in Fig. 7 show this effect for the net water-year precipitation reconstruction in the VEPIIN and VEPIIS study areas, respectively, in year AD 1400. Spatial artefacts tend to be less extreme in the GDD reconstruction, as temperature is a far less local phenomenon than precipitation in our study areas. Still, such artefacts impact the size and extent of the maize growing niche reconstruction at annual timescales, and often lead to unlikely spatial configurations of the maize niche (although these artefacts generally disappear when the reconstruction is averaged over larger timescales). 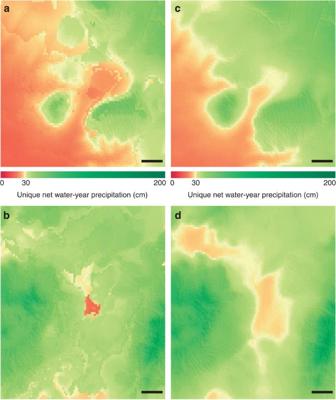Figure 7: Spatial artefacts and chronology standardization. These maps present spatial net water-year precipitation reconstructions in AD 1400 using cell-wise unique CAR selection (left panels) and the union of selected chronologies (right panels) across each study area. The cell-wise unique reconstructions show spatial artefacts because of inconsistencies between regional tree-ring chronologies. Using the union of all sets of selected tree-rings ameliorates these inconsistencies, although at a slight loss of cell-wise model performance. Scale bar, 10 km. (a) VEPIIN, unique reconstructions. (b) VEPIIS, unique reconstructions. (c) VEPIIN, union reconstructions. (d) VEPIIS, union reconstructions. Figure 7: Spatial artefacts and chronology standardization. These maps present spatial net water-year precipitation reconstructions in AD 1400 using cell-wise unique CAR selection (left panels) and the union of selected chronologies (right panels) across each study area. The cell-wise unique reconstructions show spatial artefacts because of inconsistencies between regional tree-ring chronologies. Using the union of all sets of selected tree-rings ameliorates these inconsistencies, although at a slight loss of cell-wise model performance. Scale bar, 10 km. ( a ) VEPIIN, unique reconstructions. ( b ) VEPIIS, unique reconstructions. ( c ) VEPIIN, union reconstructions. ( d ) VEPIIS, union reconstructions. Full size image In order to remove the visible spurious spatial artefacts before modelling the maize growing niche, we perform data standardization across both study areas on an annual basis. For each year (AD 1–2000), we first take the union of all sets of cell-wise-selected t-r chronologies across the landscape. Doing this for each year creates a new sequence of selected chronologies that is the spatiotemporal union of each of the unique reconstructions. We then calibrate new sequences of shrinkage linear models for each cell on the landscape, using these union sets of t-r chronologies and the original shrinkage intensities calculated above. This smooths our spatiotemporal reconstructions at a slight loss to model performance across the landscapes. Reduction in model performance generally increases through time, as locations across the landscapes begin selecting a larger union set of t-r chronologies, thus slightly overfitting models across the landscape. This solution—annual chronology standardization across each landscape by taking the union of selected proxy signals—is obviously somewhat ad hoc , and its negative impact on reconstruction skill will increase with the size or heterogeneity of the landscape. We offer it as a solution intermediate between the a priori selection of proxies common in spatial paleoclimate reconstruction today, and not correcting spatial artefacts at all. Shrinkage estimation of regression coefficients Once the RMSE-optimized and annually unioned set of t-r chronologies have been selected, we calculate regression coefficients by least squares regression of climate signal in each cell on the selected t-r chronologies over the 1924–1983 period, again using the shrinkage estimates of the covariance and correlation matrices calculated previously (applying λ υ and λ c ). Mean and variance matching over the calibration period By design, prediction using multiple linear regression reduces the variance of a reconstructed signal to the proportion of the variance in the calibration signal explained by the predictors. This has the effect of shrinking the variance over the reconstruction and, in the case of climate reconstructions where the number of available predictor variables decreases as you go farther back in time, creates a reconstruction with (generally) monotonically increasing variance. To correct this, we transform and scale each reconstruction such that the mean and variance of the reconstruction over the calibration period matches the mean and variance of the calibration data set. The transformation (mean-matching) and scaling (variance-matching) parameters are thus calculated only over the calibration period, then applied over the whole of the reconstruction. Let X c be the vector of calibration values over the calibration period, X r be the vector of reconstructed values over the calibration period, A r be the vector of all reconstructed values (of which X r is a part) and vector of all reconstructed values after mean and variance matching. Then, where, or a scalar that is the ratio of the standard deviations of the calibration and reconstructed vectors over the calibration period, and, or a transformation to the mean of the calibration vector corrected by the scaled mean of the reconstructed data over the calibration period. Thus, every reconstruction for a particular cell will have the same mean and variance over the calibration period. Retrodiction over all available data Our reconstruction proceeds in a stepwise manner backwards, starting with the calibration period and ending at the first year of the reconstruction period (here, AD 1). At each step, a reconstruction is made that extends as far back in time as all selected t-r chronologies will allow. At the year when one of the selected chronologies drops out of the sequence, RMSE selection, landscape-wide chronology standardization and shrinkage estimation of the regression coefficients are repeated with the remaining available chronologies, but still using the original CAR ranking of chronologies. Thus, a new reconstruction is not completed at every change in the t-r chronology set (see Fig. 6 ), but only when t-r chronologies deemed important by the ranking and selection process are no longer available. This retrodiction process yields an optimized (in terms of computational time) set of sequential reconstructions; each reconstruction begins at the earliest year when all its selected t-r chronologies are available, and ends at the beginning of the subsequent reconstruction. Model performance through time We used threefold consecutive (adjacent) cross-validation over the 1924–1983 period to generate fit statistics for each RMSE-minimized model. This differs from the twofold sequential cross-validation usually performed in paleoclimate research [1] , [50] , which generate reconstructions over a calibration data set and withhold a portion of historic data for model validation. Although the PRISM data set extends back to 1895, it has a well-documented increase in uncertainty before 1924 that makes the use of the 1895–1923 data as a validation data set inappropriate. The statistics presented here are averaged over the three folds; each fold calibrates with 40 years of data, and validates with the remaining 20 (for example, calibrating with 1944–1983, and validating with 1924–1943). Reconstruction skill Model performance is measured on an annually resolved cell-wise basis using three important performance statistics: The validation , the normalized RMSE (RMSE n ) and the coefficient of efficiency (CE) [1] , [3] (see Supplementary Methods for descriptions of each measure). 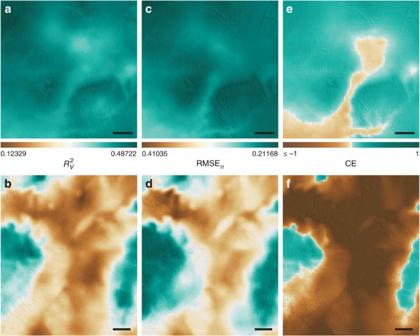Figure 8: Model skill in reconstructing net water-year precipitation. Values shown are averaged over the entire 2,000-year reconstruction., validationR2; RMSEn, normalized root mean squared prediction error; CE, coefficient of efficiency. Each performance statistic has its own legend and colour scale. Scale bar, 10 km. (a) VEPIIN. (b) VEPIIS. (c) VEPIIN RMSEn. (d) VEPIIS RMSEn. (e) VEPIIN CE. (f) VEPIIS CE. Figure 8 shows these averaged over the entire 2,000-year net water-year precipitation reconstruction, and Fig. 9 shows the same for the growing-season GDD reconstruction. It should be noted that due to the nonlinear trend in t-r chronology availability ( Fig. 6 ), these temporally averaged measures are a poor reflection of model performance, especially for reconstructions during the last millennium (see Supplementary Movies 2 and 3 for maps of reconstruction skill through time). Still, we can make several observations. Precipitation reconstructions ( Fig. 8 ) generally perform better for high-elevation (and thus higher-precipitation) locations; reconstructions at these locations are not only better-correlated with withheld cross-validation data, but also generate reconstructions with lower proportional prediction error. A somewhat different pattern exists in the GDD reconstructions ( Fig. 9 ); and RMSE n are highest in mid-elevations on portions of the landscape with consistent gradients. Drainages, including the major river valleys of the Rio Grande and Chama rivers in the VEPIIS study area, perform well, as does the Mesa Verde cuesta. Figure 8: Model skill in reconstructing net water-year precipitation. Values shown are averaged over the entire 2,000-year reconstruction. , validation R 2 ; RMSE n , normalized root mean squared prediction error; CE, coefficient of efficiency. Each performance statistic has its own legend and colour scale. Scale bar, 10 km. ( a ) VEPIIN . ( b ) VEPIIS . ( c ) VEPIIN RMSE n . ( d ) VEPIIS RMSE n . ( e ) VEPIIN CE. ( f ) VEPIIS CE. 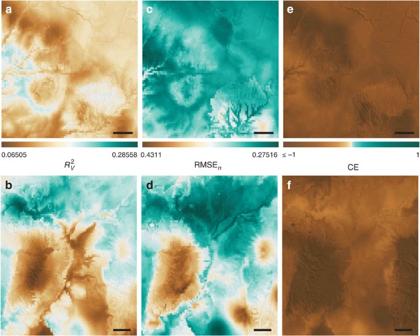Figure 9: Model skill in reconstructing growing-season growing degree days. Values shown are averaged over the entire 2,000-year reconstruction., validationR2; RMSEn, normalized root mean squared prediction error; CE, coefficient of efficiency. Each performance statistic has its own legend and colour scale. Scale bar, 10 km. (a) VEPIIN. (b) VEPIIS. (c) VEPIIN RMSEn. (d) VEPIIS RMSEn. (e) VEPIIN CE. (f) VEPIIS CE. Full size image Figure 9: Model skill in reconstructing growing-season growing degree days. Values shown are averaged over the entire 2,000-year reconstruction. , validation R 2 ; RMSE n , normalized root mean squared prediction error; CE, coefficient of efficiency. Each performance statistic has its own legend and colour scale. Scale bar, 10 km. ( a ) VEPIIN . ( b ) VEPIIS . ( c ) VEPIIN RMSE n . ( d ) VEPIIS RMSE n . ( e ) VEPIIN CE. ( f ) VEPIIS CE. Full size image Aggregating model performance spatially presents a somewhat more useful assessment of model fit. 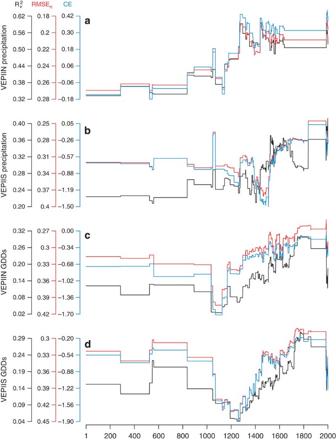Figure 10: Reconstruction skill through time. , validationR2; RMSEn, normalized root mean squared prediction error; CE, coefficient of efficiency; GDDs, growing-season growing degree days. Note the inverted scale for RMSEn. (a) VEPIIN precipitation. (b) VEPIIS precipitation. (c) VEPIIN GDDs. (d) VEPIIS GDDs. Figure 10 presents time series of model performance for the net water-year precipitation and growing-season GDD reconstructions, respectively. Model performance generally improves through time in both reconstructions, especially after AD 1200. That being said, neither study area achieves average CE values >0 during the GDD reconstructions, although this measure could very well be influenced by the skewed nature of the CE metric. Figure 10: Reconstruction skill through time. , validation R 2 ; RMSE n , normalized root mean squared prediction error; CE, coefficient of efficiency; GDDs, growing-season growing degree days. Note the inverted scale for RMSE n . ( a ) VEPIIN precipitation. ( b ) VEPIIS precipitation. ( c ) VEPIIN GDDs. ( d ) VEPIIS GDDs. Full size image The CAR method is highly effective in selecting t-r chronologies appropriate to each location and climate signal and that reflect well-documented regional climate patterns and medium-range teleconnections ( Supplementary Methods ; Supplementary Figs 4 and 5 ). Furthermore, CAR reconstructions over the historic period show prediction skill comparable to or better than the PCR method used in the North American Drought Atlas [1] , [2] , [3] , and greatly outperform reconstructions that use the marginal correlation for variable ranking ( Supplementary Methods ; Supplementary Table 17 ). Uncertainty estimation Uncertainty in the size of the rain-fed maize agricultural niche is a function of the compound error in the PRISM weather interpolations, t-r measurement and signal noise, and cell-wise CAR reconstructions. A full description and quantification of each of these sources of uncertainty are beyond the scope of this paper. However, to aid in interpretation we define a first-order approximation of the prediction interval (PI) for each cell i in each year t as, where x is the predicted value, and RMSE is the cross-validated RMSE for the cell’s linear model. This generates annual prediction intervals for each cell for both the precipitation and GDD reconstructions. We derive prediction intervals for the spatial extent of the rain-fed maize agricultural niche by overlaying the lower and upper intervals for each climate signal ( Fig. 3 , Supplementary Movie 1 ). These prediction intervals do not incorporate uncertainty in the PRISM weather interpolations or uncertainties stemming from t-r measurement and signal noise. Spatial uncertainty estimates for the LT81m PRISM data set used in this study have not been published; estimates for an earlier version of the PRISM data set (‘LT71m’) are presented by Daly and colleagues [41] . Examples and model comparison The online Supplementary Information presents local paleoclimate reconstructions at four weather stations across the SWUS as an example of the CAR method ( Supplementary Methods ; Supplementary Figs 2–5 ; Supplementary Tables 1–17 ). These four reconstructions are then compared with those produced using the PPR method from the North American Drought Atlas [1] , [2] , [3] , [50] and those produced by ranking chronologies by their marginal correlations with the local climate signal. How to cite this article: Bocinsky, R. K. et al. A 2,000-year reconstruction of the rain-fed maize agricultural niche in the US Southwest. Nat. Commun. 5:5618 doi: 10.1038/ncomms6618 (2014).